Neuroplasticity-based computerized cognitive remediation for treatment-resistant geriatric depression Executive dysfunction (ED) in geriatric depression (GD) is common, predicts poor clinical outcomes and often persists despite remission of symptoms. Here we develop a neuroplasticity-based computerized cognitive remediation-geriatric depression treatment (nCCR-GD) to target ED in GD. Our assumption is that remediation of these deficits may modulate the underlying brain network abnormalities shared by ED and depression. We compare nCCR-GD to a gold-standard treatment (escitalopram: 20 mg per 12 weeks) in 11 treatment-resistant older adults with major depression; and 33 matched historical controls. We find that 91% of participants complete nCCR-GD. nCCR-GD is equally as effective at reducing depressive symptoms as escitalopram but does so in 4 weeks instead of 12. In addition, nCCR-GD improves measures of executive function more than the escitalopram. We conclude that nCCR-GD may be equally effective as escitalopram in treating GD. In addition, nCCR-GD participants showed greater improvement in executive functions than historical controls treated with escitalopram. Despite significant developments, conventional antidepressant treatments leave many older adults depressed and suffering [1] . Antidepressants developed in the past 20 years are safe but their efficacy is no better than that of tricyclics. The onset of antidepressant action is slow, improvement of symptoms is often incomplete and unstable, and remission occurs in only one-third of patients [2] . In addition, if the patient suffers from ED, they are almost two times less likely to respond to medications [3] , [4] . Psychotherapy may be effective in some depressed elders, although a recent review concluded that none of the available treatment studies met stringent criteria for efficacy in the acute treatment of geriatric depression (GD) [5] . The recent National Institute of Mental Health report ‘From Discovery to Cure’ calls for studies focusing on mechanisms of treatment response with the goal of arriving at new interventions for those who do not respond to existing treatments. It is in response to this report and our group’s previous findings that we developed a treatment designed to change the functioning of a cerebral network, we and others have found associated to be with poor treatment response in GD [6] , [7] , [8] , [9] , [10] . Replicated studies document that ED in geriatric depressed patients leads to adverse clinical outcomes including poor and slow response to antidepressants [11] , [12] , [13] , [14] , [15] , [16] , [17] , [18] , disability [19] , increased risk for relapse [20] and suicidal ideation [21] . In addition, ED often persists despite remission of mood symptoms [6] , [22] , [23] , leaving patients perpetually vulnerable. Within executive functions, susceptibility to cognitive interference, and impairment in strategic semantic organization are two functions that have repeatedly been linked to poor remission rates independently of processing speed [8] , [14] , [15] , [24] , [25] . Last, more than 40% of elderly depressed patients suffer from ED [26] , making it a common dysfunction, that if successfully treated, could significantly improve the treatment outcomes of late-life depression [27] . Recent findings from both human [28] , [29] , [30] , [31] and animal [32] studies suggest that the aging brain can make neuroplastic changes with enhanced activity [33] , [34] . Neuroplasticity-based computerized cognitive remediation (nCCR) has been shown to reverse age-related declines in information encoding and processing, and induce change in the underlying neural functions [29] , [30] . In older adults, nCCR improves basic cognitive functions such as memory [31] and processing speed [31] , as well as executive functions such as cognitive control [28] , task shifting, resolving interference [35] and dual-task processing [36] . Further, nCCR training ‘generalizes’ and induces both proximal and distal transfer [31] , [36] . Effects of nCCR are also sustainable, with benefits remaining at least 3 months after training [30] . Finally, nCCR appears to induce changes on measures of ‘neuroplasticity’ in the aging brain. nCCR-induced changes in brain structure and function [37] , [38] , [39] in the elderly are similar to neurobiological effects in young adults, and correlate with improvements in cognitive performance [38] , [40] . Encouraged by the specificity of our cognitive findings, we designed nCCR-GD. We based the basic principles of nCCR-GD on the theory that neuroplasticity in an aged brain requires intensive practice coupled with the heightened neurotransmission associated with reward (modulated by dopamine and norepinephrine) [41] . To meet this goal, we designed nCCR-GD behavioural-training paradigms to engage targeted cerebral networks with sensory, motor and cognitive tasks that are: (1) increasingly challenging; (2) individually adaptive; (3) attention demanding; and (4) immediately rewarding. nCCR-GD was designed to train depressed older adults on the specific executive functions that predict treatment response in GD (that is, cognitive inhibition [14] , [25] , [42] verbal strategy initiation and utilization [3] , [4] , as well as aspects of cognitive control that rely on overlapping networks (that is, cognitive flexibility, set shifting, inhibition of prepotent responses). We aimed to target the cerebral networks (including dorsolateral prefrontal cortex, orbitofrontal cortex, dorsal anterior cingulate cortex) associated with these executive functions. Our selection of behavioural-training paradigms to target executive functions for nCCR-GD was informed by other nCCR studies in normal older adults that demonstrated successful remediation of target executive deficits due to normal aging [29] , [38] , [43] . Our preliminary findings suggest that nCCR-GD may be equally effective as escitalopram in treating the affective symptoms of GD. In addition, nCCR-GD participants show greater improvement in clinically relevant executive functions than those treated with escitalopram alone. As a first step, we tested this intervention with depressed older adults who had failed at least one trial of an antidepressant (selective serotonin reuptake inhibitor or serotonin–norepinephrine reuptake inhibitor) at an adequate dose for at least 8 weeks. The objectives of this study were: (1) to test the feasibility of this novel treatment modality in a geriatric depressed sample, (2) to compare our treatment (nCCR-GD for 4 weeks) to a control, gold-standard treatment (escitalopram; target dose:20 mg for 12 weeks). This study tests the hypothesis that nCCR-GR offered to geriatric patients with major depression who had failed at least one adequate antidepressant (selective serotonin reuptake inhibitor or serotonin–norepinephrine reuptake inhibitor) trial will improve on measures of both executive functioning and depression more than those taking escitalopram alone. We also hypothesized that the nCCR-GD would improve not only the functions trained by the programs, but generalize to other executive functions that rely on networks similar to the targeted network (‘near-transfer’). CCR-GD versus escitalopram Of the 11 participants, 10 completed the 4-week treatment (91%). 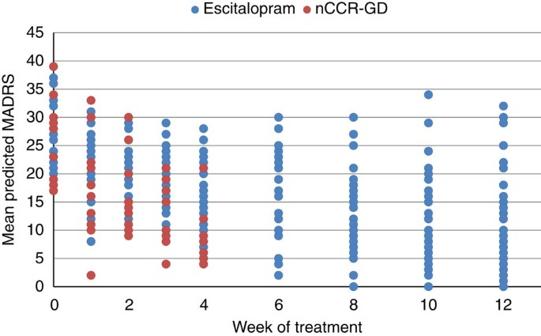Figure 1: Participant data: Depression severity by week of treatment. Depiction of participants’ depression scores on the Montgomery–Asberg Depression Rating Scale (MADRS) by each week of treatment. Twelve weeks for the escitalopram group and 4 weeks for the nCCR-GD group. At baseline, there were no differences (escitalopram versus nCCR-GD) in Montgomery–Asberg Depression Rating Scale (MADRS) ( U =180.0, P =0.967), in age ( U =173; P =0.818), education ( U =141.5; P =0.273), age of onset ( U =153; P =0.440) or executive function (Trails B) ( U =152; P =0.424) ( Table 1 ). Table 1 Baseline participant characteristics. Full size table Mixed effects model analysis showed no significant group main effect ( F (1,49.23)=0.019, P =0.892). However, the time effect ( F (1,71.22)=30.97, P <0.001) and treatment group × time interaction ( F (1,61.8)=5.32, P =0.024) reached significance indicating that the slope of MADRS decline was steeper in the nCCR-GD group ( Figs 1 and 2 ). At the end of 4 weeks of treatment, the mean MADRS score in the nCCR-GD group was 8.9 (s.d.=4.8), lower ( t =3.052; df=38; P =0.004) than the escitalopram group mean score 15.5 (s.d.=6.1). Figure 1: Participant data: Depression severity by week of treatment. Depiction of participants’ depression scores on the Montgomery–Asberg Depression Rating Scale (MADRS) by each week of treatment. Twelve weeks for the escitalopram group and 4 weeks for the nCCR-GD group. 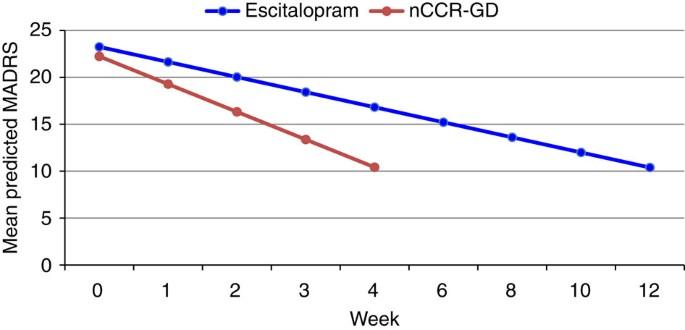Figure 2: Mixed models predicted values. Efficacy (MADRS score over time) of treatment groups was compared with longitudinal mixed models analysis with a random intercept and time (weeks from baseline), treatment group, and a time by treatment group interaction as fixed effects. Full size image Figure 2: Mixed models predicted values. Efficacy (MADRS score over time) of treatment groups was compared with longitudinal mixed models analysis with a random intercept and time (weeks from baseline), treatment group, and a time by treatment group interaction as fixed effects. Full size image nCCR-GD improved Trails B performance more than escitalopram ( t =2.28, df=41; P =0.027) ( Fig. 3 ); and there was a trend for the Stroop Color-Word ( t =1.86, df=41; P =0.103) ( Fig. 4 ). 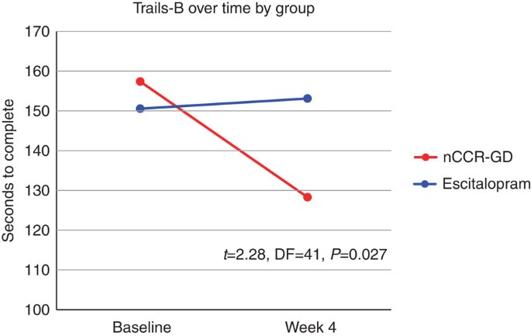Figure 3: Changes in time to complete trails B over time by group. Depiction of the change from baseline to post treatment in participants treated with escitalopram and participants treated with nCCR-GD on the Trail Making Test part B, a test of executive function measuring cognitive flexibility. Figure 3: Changes in time to complete trails B over time by group. Depiction of the change from baseline to post treatment in participants treated with escitalopram and participants treated with nCCR-GD on the Trail Making Test part B, a test of executive function measuring cognitive flexibility. 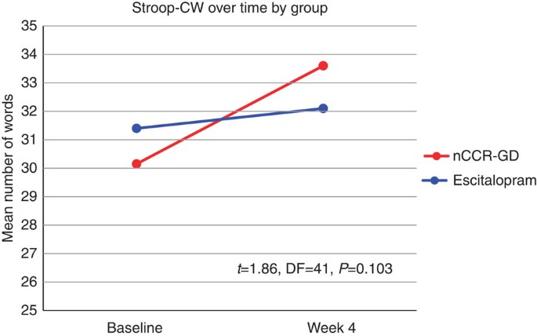Figure 4: Changes in Stroop Color-Word over time by group. Depiction of the change from baseline to post treatment in participants treated with escitalopram and participants treated with nCCR-GD on the Stroop Color-Word, a test of executive function measuring inhibition of prepotent responses. Full size image Figure 4: Changes in Stroop Color-Word over time by group. Depiction of the change from baseline to post treatment in participants treated with escitalopram and participants treated with nCCR-GD on the Stroop Color-Word, a test of executive function measuring inhibition of prepotent responses. Full size image nCCR-GD response rates Of the 11 patients, 9 patients met criteria for response to treatment at the end of 4 weeks. At the 12-week no-contact follow-up, 6 of 11 patients met criteria for response to treatment. nCCR-GD remission rates After 4 weeks, 8 of the 11 patients met criteria for remission [44] . At the 12-week follow-up, 6 of 11 patients met criteria for remission. Neurocognitive change in the nCCR-GD group In the nCCR-GD group, we conducted exploratory analysis of change in performance from baseline to treatment end (paired t -tests) on targeted as well as transfer of benefit to non-targeted executive functions, and to distal cognitive functions that rely on intact performance of executive functions. There was an improvement in performance on the Stroop Color-Word ( t =−3.051; df=9; P =0.014), Trails B ( t =3.554; df=9; P =0.024) and design fluency-switching on the Delis Kaplan Executive Functioning System (DKEF-S) ( t =−4.243; df=9; P =0.002). There was a trend for semantic clustering on the Mattis Dementia Rating Scale Initiation/Perseveration (DRS I/P) ( t =−2.236; df=9; P =0.052), that is, participants may have increased the number of semantic clusters they used to complete the DRS I/P. There was no pre- to post-nCCR-GD treatment difference in performance in working memory (Wechsler Adult Intelligence Scale-fourth Edition (WAIS-IV) digits backwards ( t =0.197; P =0.849)); or in verbal memory (California Verbal Learning Test Second Edition (CVLT-ii) long delay recall ( t =1.00; P =0.347)). There was a correlation between improvements in Trails B performance before and after CCR-GD treatment with improvements in MADRS scores (Spearman’s r =0.723; P =0.018), but not between improvements in the Stroop and improvements in MADRS scores (Spearman’s r =0.096; P =0.560). 12-Week follow-up after completion of nCCR-GD Depressive symptoms: there was no significant difference in participants’ MADRS scores from treatment completion (week 4) to follow-up 12 weeks later ( t =−0.505; df=9; P =0.626). Cognitive scores: there was no difference between scores on Stroop Color-Word ( t =−1.155; P =0.30), Trails B ( t =0.379; P =0.720), semantic clustering ( t =−1.00; P =0.356), digits backwards ( t =0.444; P =0.673); CVLT-ii Long delay recall ( t =1.035; P =0.348) or design fluency-switching ( t =−0.573; P =0.587) from the end of the treatment trial (4 weeks), to assessment at the 12-week follow-up. These results suggest that the initial improvement in depressive symptoms as well as the neurocognitive gains made by nCCR-GD were sustained for at least 12 weeks (3 months) post treatment. The principal finding of this study is that nCCR-GD is feasible and equally effective with escitalopram in older adults with major depression. Ten of the 11 study participants completed the trial as prescribed. When compared with escitalopram treatment, nCCR-GD reduced MADRS scores to the same level in four as opposed to 12 weeks. Moreover, participants in the nCCR-GD group were classified as treatment resistant; all had failed at least one adequate trial of an antidepressant. The escitalopram group was not similarly selected for treatment-resistant participants. This is the first study, to our knowledge, to document that an nCCR intervention targeting executive and related network functions can improve both mood and cognitive functions in drug-resistant, late-life depression. In addition to the reduction in depression scores, nCCR-GD appeared to improve executive functions more than escitalopram; the nCCR-GD participants’ improved scores on a measure of cognitive flexibility (Trails B) over the treatment trial more than the escitalopram group, there was a trend for improvement of inhibiting prepotent responses (Stroop Color-Word). This finding is of particular clinical significance as elderly patients with ED are less likely to remit using conventional antidepressants. In addition, even if the depressive syndrome subsides, antidepressants are unlikely to improve executive deficits leaving them perpetually vulnerable to disability and relapse. Further, our hypotheses regarding the cognitive benefits of nCCR-GD were confirmed. The nCCR-GD group exhibited improved cognitive performance on targeted executive functions. Near-transfer of benefit was also observed in non-targeted but related executive functions. However, transfer to more distal cognitive functions (that is, verbal memory, working memory) that rely on intact performance of executive functions did not improve post treatment. If these cognitive benefits are replicated, improved executive functioning through nCCR-GD may increase both the number of patients who are able to reach remission, as well as the number who are able to sustain prolonged remission. Last, both affective and cognitive benefits observed from participation in nCCR-GD were sustained at least 3 months post completion. The sustainability of neurocognitive gains in our population is equivalent to those seen in other nCCR trials in normal aging [45] . There are several important limitations that have variable impacts on the results of this preliminary study. We, therefore, encourage an appropriately tempered interpretation of these findings. The first is the study’s small sample size. Given the small number of participants in this pilot trial, we can only speculate as to the generalizability of this finding. Second and perhaps most significant is the lack of an active, concurrently studied control group. The historical comparator group may not be an adequate comparison group due to multiple factors including the difference in duration, modality and trial type. In addition to these effects, a control treatment provided in the same modality (computer) will be necessary to decipher whether targeted nCCR-GD is necessary to induce change in mood and cognitive symptoms of GD, or whether similar results could be achieved by non-specific stimulation. This last point is essential to the investigation of our hypothesis that targeting specific, and clinically relevant circuitry related to the pathophysiology of the illness is key to inducing both cognitive and affective change. Third, is the lack of prospective random assignment of subjects to the active and control groups. Though the groups were matched on clinically relevant variables, there are significant differences between the two groups, for example, they were not similarly selected for prior treatment failure. Last, assessing neuropsychological performance before and after treatment required that some measures be repeated. Given that the treatments (escitalopram versus nCCR-GD) differed in length, it is possible that the difference in scores may be partially explained by a practice effect. However, 7 of the 10 nCCR-GD participants had already undergone the escitalopram trial and experienced the tests before entry to nCCR-GD. This is a preliminary study conducted to test the feasibility of an nCCR in an elderly depressed population. Future iterations of this investigation will include larger samples randomized either to nCCR-GD or a concurrently studied, computer-presented control condition. There are several control treatment options worth considering. For example, the use of a pre-packaged, non-targeted CCR intervention, a nCCR intervention targeted to a different neural circuit, or an equally stimulating computer activity. A larger sample will allow for further investigation of the targeted neural circuits in the pathogenesis of GD as well as their relationship to treatment response by answering (for example): if changes in executive function induced by nCCR-GD are related to changes in depressive symptoms? ; if ED at baseline is a moderator of treatment response? ; whether targeting other circuitry achieves similar results or if this result is only achieved with specificity in target selection? nCCR-GD was designed to be mutable as well as to give incremental feedback to investigators about whether the programs are performing as designed. As cognitive and affective neuroscience progresses, nCCR designs can progress in parallel, with new discoveries serving as targets for newly developed nCCR protocols. In conclusion though the data are preliminary, nCCR-GD appears improve affective symptoms more quickly than escitalopram in patients who have previously failed to respond to pharmacotherapy. In addition, nCCR-GD may improve both targeted and non-targeted executive functions while escitalopram does not. Participants nCCR-GD participants were older adults (60–89) with major depression (by SCID-R/DSM-IV), who failed to achieve remission (MADRS>15) after treatment with therapeutic dosages of an selective serotonin reuptake inhibitor or serotonin–norepinephrine reuptake inhibitor antidepressant for at least 8 weeks ( Fig. 5 ). In addition, we asked that they and their physicians had no plan to change medication or dosages for the duration of the study (4 weeks) unless required by significant worsening of clinical symptoms. 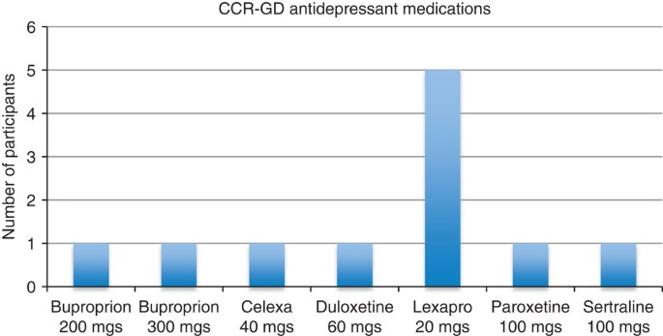Figure 5: CCR-GD participant antidepressant medications. Depiction of the antidepressant medications taken for at least 8 weeks by nCCR-GD participants throughout the 4 weeks of treatment. No participant changed their medications or dosages throughout the study. Figure 5: CCR-GD participant antidepressant medications. Depiction of the antidepressant medications taken for at least 8 weeks by nCCR-GD participants throughout the 4 weeks of treatment. No participant changed their medications or dosages throughout the study. Full size image Weill Cornell Medical College Institutional Review Board reviewed and approved all procedures. In total, 11 of 12 patients who met criteria and were approached signed informed consent and entered the study (mean age=73.5 years; s.d.=7.8). The sample was 63.6% female, 36.4% male. In total, 8 of 11 participants were recruited after failing to remit during a controlled 12-week escitalopram trial (target dose 20 mg). The other three participants were referred to the study by their psychiatrists after failing multiple trials of antidepressants. Of the 11 patients, 10 completed the 4-week trial. One patient dropped at week 2 due to an inability to maintain the required frequency of clinic visits. All participants were questioned weekly about any changes to their medications; all maintained the same medication and dosage throughout the treatment period. Participants underwent a neuropsychological battery at baseline, after 4 weeks of treatment, and 12 weeks post completion of nCCR-GD (week 16). All participants met DSM-IV-TR criteria and Research Diagnostic Criteria for unipolar major depression and had a MADRS score >15. Exclusion criteria were: (1) major depression with psychotic features (according to DSM-IV-TR); (2) history of other psychiatric disorders (except personality disorders) before the onset of depression; (3) severe medical illness (that is, metastatic cancer, brain tumours, unstable cardiac, hepatic or renal disease, myocardial infarction or stroke) within the 3 months preceding the study; (4) neurological disorders (that is, dementia or delirium according to DSM-IV criteria, history of head trauma, Parkinson’s disease and multiple sclerosis); (5) conditions often associated with depression (that is, endocrinopathies other than diabetes, lymphoma and pancreatic cancer); (6) drugs causing depression (that is, steroids, α-methyl-dopa, clonidine, reserpine, tamoxifen and cimetidine); and (7) Mini-Mental State Examination [46] score <25 or Mattis Dementia Rating Scale scores below 130; (8) amnestic or multiple-domain mild cognitive impairment; (9) current psychotherapy; (10) inability to speak English (nCCR-GD games are in English only); corrected visual acuity <20/70 or colour blindness. These criteria resulted in a group of elderly patients with non-psychotic unipolar major depression without a diagnosable dementing disorder. Comparison escitalopram participants Escitalopram participants included 33 matched (three escitalopram participants to each nCCR-GD participant) depressed, elderly (>60 years) patients from a university-based geriatric psychiatry clinic who were recruited for a 12-week escitalopram treatment trial. Each historical control was matched on three criteria: age, depression severity and ED (Stroop CW performance). We chose these criteria due to their demonstrable effect on clinical outcomes in GD. Neuropsychological tests were performed during a 2-week single blind psychotropic drug wash-out/placebo lead-in phase, and after 12 weeks of treatment. Escitalopram participants met DSM-IV-TR criteria and Research Diagnostic Criteria for unipolar major depression and had a score >19 on the 24-item Hamilton Depression Rating Scale [47] . Exclusion criteria were: (1) major depression with psychotic features (according to DSM-IV-TR); (2) history of other psychiatric disorders (except personality disorders) before the onset of depression; (3) severe medical illness (that is, metastatic cancer, brain tumours, unstable cardiac, hepatic or renal disease, myocardial infarction or stroke) within the 3 months preceding the study; (4) neurological disorders (that is, dementia or delirium according to DSM-IV criteria, history of head trauma, Parkinson’s disease and multiple sclerosis); (5) conditions often associated with depression (that is, endocrinopathies other than diabetes, lymphoma and pancreatic cancer); (6) drugs causing depression (that is, steroids, α-methyl-dopa, clonidine, reserpine, tamoxifen and cimetidine); and (7) Mini-Mental State Examination [46] score <25; (8) current psychotherapy. These criteria resulted in a group of elderly patients with non-psychotic unipolar major depression without a diagnosable dementing disorder. Side effects of escitalopram were monitored with the Udvalg for Kliniske Undersøgelser side-effect scale [48] . Control escitalopram treatment Patients were informed that they would receive placebo at some point during their 14-week trial. After a 2-week psychotropic drug wash-out and single blind placebo lead-in, subjects who still met DSM-IV-TR criteria for major depression and had a 24-item Hamilton Depression Rating Scale score of 19 or greater received controlled treatment with escitalopram (target dose 20 mg) daily for 12 weeks. Patients were instructed to take a single dose of escitalopram in the morning, and were administered medication in 1-week supply blisters that permitted dispensation of their daily dosage separately. The treatment phase consisted of weekly follow-up sessions beginning with the placebo lead-in, continuing until the 12th week of treatment with escitalopram. During each follow-up meeting, a research assistant administered the Hamilton Depression Rating Scale, MADRS, the Udvalg for Kliniske Undersøgelser, obtained vital signs, questioned the subjects about medication adherence and counted the remaining tablets. This meeting was followed by a brief session with a research psychiatrist to assess the risk of continuing the treatment trial and to clinically confirm any remission. The session followed a medication clinic model consisting of a review of symptoms, explanations related to the need for treatment and encouragement of treatment adherence. No subject received psychotherapy during the study. nCCR-GD Participants completed 30 h of cognitive remediation over 4 weeks on computer stations in private treatment rooms at the Advanced Center for Interventions and Services Research. The brief 4-week time period was chosen to mitigate several factors: The selected participants were treatment resistant and quite symptomatic; CCR-GD was an as-yet-untested treatment and participants were continuing to take a dose of medication that was ineffective. Participants had access to the supervising psychologist and research assistants for questions at any time, but after the initial programme set up, participants worked on their own without intervention. Three ‘Bottom Up’ training exercises were used: one low-level auditory tone sweep and one phonemic discrimination task from ‘Brain Fitness’ and one low-level visual discrimination training exercise from ‘Insight’ [45] , [49] . These programs were designed for older adults to enhance basic processing of sensory stimuli with the goal to improve fidelity of initial auditory and visual encoding [31] , [45] , [49] . ‘Top Down’ training exercises were newly developed by our group and incorporated into two user interfaces. The first is ‘Catch the Ball’ (individually titrated training in visual attention, inhibition of prepotent responses, working memory, cognitive flexibility and dual-task performance). Participants view moving balls on a blue screen and are instructed to press the button when the ball turns to a target colour. Balls change from yellow to the target or foil colour (blue, red, green) at random intervals (1.5–3.5 s). Initial difficulty levels focus on sustained attention, balls simply turn to the target colour of red, with the duration of the target colour progressively decreased to increase difficulty. Next levels introduce blue foils to require discriminatory attention and response inhibition. Next, response inhibition demands are increased and cognitive flexibility introduced by having the target switch back and forth between red and blue at random intervals. All variations are then repeated first with two balls on the screen and then with three to increase overall demand, and add divided attention demands. Speed at which the balls move is adaptively tracked. Subjects are moved from one difficulty level to the next when they demonstrate sustained accuracy at the fastest ball speed or when they fail to show continued performance at a slower speed. ‘Semantic Strategy’: training in recognition and initiation of semantic strategy. Participants are asked to rearrange multiple, increasingly complex word lists into categories with individually titrated decreases in allotted processing time. Task demands increase further by including components of ‘cognitive control’, using previous sort stimuli as proactive interference. Both speed and accuracy are adaptively tracked. Training task parameters were set to keep performance between 75 and 85% correct; a balance between challenge and reward that in animal studies seems optimal for producing neuroplastic change. Participants selected the duration of sessions and a weekly schedule most desirable to them [50] . nCCR-GD programs give immediate auditory/visual rewards for correct responses [51] , and employ adaptive tracking of task difficulty in order to minimize frustration due to incorrect responses [45] as well as keeping performance levels in the desired range. The Weill Cornell Medical College Institutional Review Board approved all procedures. After a complete description of the study to subjects, written informed consent was obtained. Outcome measures Advanced Center for Interventions and Services Research-trained research assistants unaware of the study’s hypotheses collected clinical ratings, neuropsychological tests and self-report measures under the supervision of a neuropsychologist (S.S.M.). Depressive symptoms were assessed using the 10-item MADRS. Disability was measured with the World Health Organization Disability Assessment Schedule-II. Baseline gross cognitive status was rated with the Mini-Mental State Examination [46] . ‘Response’ was defined as a 50% reduction in overall MADRS from baseline to end of treatment. ‘Remission’ was defined as a MADRS score of 10 or less [44] . Neuropsychological measures: overall cognitive dysfunction was assessed with the Mattis Dementia Rating Scale. Executive functioning was assessed in both groups with two measures: inhibiting prepotent responses with the Stroop Color-Word Test [52] and cognitive flexibility with Trail Making Test B [53] . In the nCCR-GD group, we also assessed semantic clustering with semantic clusters on the Mattis Dementia Rating Scale Complex Verbal Test, verbal memory with the CVLT-ii long delay recall, non-verbal cognitive flexibility with design fluency-switching from the Delis Kaplan Executive Functioning System; and working memory with using digits backwards from the WAIS-IV. Alternate forms, where available, were used during the second administration. These tests were not administered to the escitalopram group and, therefore, scores could not be compared. Statistical analysis Baseline demographic and clinical characteristics of the two treatment groups were compared using Mann–Whitney U -statistics. Efficacy (MADRS score over time) of treatment groups was compared longitudinal mixed models analysis with a random intercept, time (weeks from baseline), treatment group, and a time by treatment group interaction as fixed effects. As nCCR-GD was designed to improve executive functions, we compared the change in executive test scores (Trails B, Stroop CW) over time (baseline, end of study) between the two treatment groups with repeated measures analysis of variances. We performed paired t -tests to compare scores on tests of executive function from baseline, to the end of nCCR-GD treatment (4 weeks) and 4 weeks to 12 weeks (or week 16 of the study) post treatment. The relationship between change in depressive symptoms and change in executive function was evaluated with Spearman’s Rho. How to cite this article: Morimoto, S. S. et al. Neuroplasticity-based computerized cognitive remediation for treatment-resistant geriatric depression. Nat. Commun. 5:4579 doi: 10.1038/ncomms5579 (2014).